Porous aromatic frameworks with anion-templated pore apertures serving as polymeric sieves Owing to environmental pollution and energy depletion, efficient separation of energy gases has attracted widespread attention. Low-cost and efficient adsorbents for gas separation are greatly needed. Here we report a family of quaternary pyridinium-type porous aromatic frameworks with tunable channels. After carefully choosing and adjusting the sterically hindered counter ions via a facile ion exchange approach, the pore diameters are tuned at an angstrom scale in the range of 3.4–7 Å. The designed pore sizes may bring benefits to capturing or sieving gas molecules with varied diameters to separate them efficiently by size-exclusive effects. By combining their specific separation properties, a five-component (hydrogen, nitrogen, oxygen, carbon dioxide and methane) gas mixture can be separated completely. The porous aromatic frameworks may hold promise for practical and commercial applications as polymeric sieves. Efficient separations of light gases (H 2 , N 2 , O 2 , CO 2 and CH 4 ) are of great concern because most of them are very important raw ingredients in the chemical and petrochemical industry [1] , [2] . At present, air separation employing cryogenic distillation, as an energy-intensive method, needs to progress urgently [3] . The capture of CO 2 also has a significant environmental impact on carbon recycling and minimizing the global warming effects [4] . Therefore, to satisfy the increasing need for a more efficient, energy-saving and environmental benign procedure, applicable adsorbents with tailored pore sizes, low cost, easy preparation and high stability must be further developed [5] . To separate gases, pore sizes among the scale range from ultramicropore (smaller than 4 Å) to micropore are all of fatal importance [6] , [7] . Attentions were focused on accurately controlling the pore sizes, which would be expected to generate precise molecular sieving discrimination [8] , [9] . As the traditional microporous materials, zeolites have been well applied in industrial catalysis, adsorption and ion exchange [10] . However, due to the limitation of types and pore diameters, there are only a few zeolites whose pores can be adjusted in a narrow range [11] . In the last decade of the twentieth century, metal–organic frameworks (MOFs), which consist of metal centres and organic ligands linked by coordination bonds, emerged as the novel porous materials [12] , [13] , [14] , [15] , [16] , [17] , [18] , [19] , [20] in gas storage [21] , [22] , [23] and separation [24] , [25] , [26] , [27] with excellent performances. The pore sizes of some MOFs can be regulated appropriately for specific gas adsorption through adjusting and modifying the ligands [28] , [29] . However, the high cost and low stability continue to be pressing problems. Recently, porous organic frameworks (POFs)—which are constituted with solely organic components and are entirely covalent in nature [30] , [31] , [32] , with lower density, high stability, crystalline structures [33] , [34] , [35] and high surface area [36] —are attracting more and more technological and scientific interests [37] , [38] . Currently, they have become the innovative organic equivalents of inorganic microporous materials with their superior properties in gas storage and separations by conditioning the pore environment [39] , [40] , [41] , [42] . Ion exchange is a feasible method to tune the channel size. One famous sample is zeolite NaA with Na + ions in cages whose pore diameters can be preciously tuned from 3 to 5 Å by ion exchange [11] . However, the classical strategy may not be suitable for most of MOFs and POFs, and there are rare works reported. And the main cause lies in the lack of necessary elements, such as right pore sizes, charged frameworks and stable skeletons. The pyridinium-type porous aromatic frameworks (PAFs), PAF-50 (named Cl-PAF-50 in this article), has organic positive charged frameworks and possesses a narrow pore size distribution centred at 5 Å close to the kinetic diameters of light gases [43] . The positive framework of Cl-PAF-50 with extra framework counter Cl − ions allows us to adjust the pore size through the exchange of Cl − to other counter ions. Here we report a series of positively charged pyridinium-type porous aromatic frameworks whose pore size can be tuned in the range of 3.4–7 Å through ion exchange with different sterically hindered counter ions. The PAFs can effectively separate the gas mixtures including H 2 , N 2 , O 2 , CH 4 and CO 2 at room temperature, as demonstrated by gas-chromatography. The series of PAFs exhibit the various interactions between the specific pore walls and gas molecules. The simple PAFs with controllable pore sizes may have wide applications as polymeric sieves. Preparation of the PAFs Positively charged quaternary pyridinium Cl-PAF-50 with counter Cl − ions has been synthesized through the condensation reaction of 4-pyridinylboronic acid and cyanuric chloride ( Supplementary Fig. 1 ) [43] . Before the ion exchange, the Cl-PAF-50 was activated under vacuum, and then washed with ethanol for several times until no free Cl − released. In the ion exchange process, tetrabutylammonium halide was added into the suspension of the Cl-PAF-50 in the anhydrous ethanol. The replacement of the sterically hindered counter ions with F − , Br − or I − ions were carried out at room temperature ( Fig. 1 ). Then, the precipitates were filtered, thoroughly washed with anhydrous ethanol and dried at 120 °C under vacuum to give F-PAF-50, Br-PAF-50 and 2I-PAF-50 powders. The tetrabutylammonium iodide was added into the ethanol solution with F-PAF-50 to give 3I-PAF-50 powders. 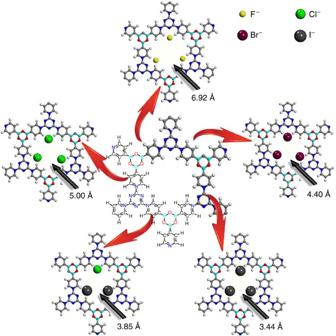Figure 1: Scheme of preparation of X-PAF-50. Scheme of preparation of F-PAF-50, Br-PAF-50, 2I-PAF-50 and 3I-PAF-50 from Cl-PAF-50. Figure 1: Scheme of preparation of X-PAF-50. Scheme of preparation of F-PAF-50, Br-PAF-50, 2I-PAF-50 and 3I-PAF-50 from Cl-PAF-50. Full size image The powder X-ray diffraction images of PAF-50s are shown in Supplementary Fig. 2 . The patterns reveal that all the samples are amorphous due to the lack of long-range ordered structures. Scanning electron microscopy (SEM) images show that the obtained PAFs are composed of aggregated particles in submicrometre sizes ( Supplementary Fig. 3 ). The Fourier transform infrared spectroscopy (FT-IR) spectra are shown in Supplementary Fig. 4 and no noticeable changes are observed about the intense B 3 O 3 bands (at 734 cm −1 ), indicating their structural integration during the ion exchange processes. The organic framework displays an excellent stability in a variety of polar and non-polar organic solvents such as acetone, ethanol, toluene and hexane. Besides, the stability of the PAF-50 against water was probed by FT-IR ( Supplementary Fig. 5 ). No noticeable spectral change was observed after 1 day soaked in water, indicating their excellent structural stability in water [43] . Ion-chromatographic analyser was used to determine the content of the halide ions exchanged in the PAFs ( Supplementary Table 1 ). The obtained data point out that the former Cl − ions were almost fully replaced with other ions including F − and Br − . For the iodic PAF-50, only about two-thirds of Cl − ions were substituted by I − using the same starting material, which was probably because the pore openings of Cl-PAF-50 were too narrow for the complete exchange. In an alternative way, the fully substituted 3I-PAF-50 is obtained by exchange I − ion with the F-PAF-50, possessing a larger pore size. Thermogravimetric analysis (TGA) suggested the weight losses of all the PAFs corresponding to the decomposition of the skeleton occurred over 220 °C, and the residual at 800 °C were 31.2, 29.0, 24.0, 21.9 and 18.89 wt% for F-PAF-50, Cl-PAF-50, Br-PAF-50, 2I-PAF-50 and 3I-PAF-50, respectively ( Supplementary Fig. 6 ). The TGA results are coincident with the content of halide ions loaded in Cl-PAF-50 calculated by the following theoretical simulation (calculated. 32.2, 28.1, 22.9, 21.2 and 17.9 wt% for F-PAF-50, Cl-PAF-50, Br-PAF-50, 2I-PAF-50 and 3I-PAF-50, respectively). Theoretical simulation The pore structures of the serial PAFs were calculated by Materials Studio (MS) simulation environment employing MS Visualizer ( Supplementary Fig. 1 ). Energy minimization optimization was performed utilizing force–field calculations to obtain reasonable bond lengths and angles. The above results indicated that the pore size of Cl-PAF-50 was about 5 Å. The diameters of charge-balancing F − , Cl − , Br − and I − ions are 2.66, 3.62, 3.92 and 4.40 Å (ref. 44 ), respectively. After substituting the Cl − with F − and Br − , F-PAF-50 and Br-PAF-50 possess the pore sizes centred at 6.9 and 4.4 Å, respectively. In addition, a replacement of the counter ions Cl − with I − would lead to ultramicroporous structure in the framework. If the exchange were fully completed, the pore size is expected to locate at 3.4 Å, and if the two-thirds of the Cl − ions were replaced, the pore dimension would be 3.9 Å. However, once the two-thirds of Cl − ions were occupied in Cl-PAF-50, the windows of 2I-PAF-50 would be too narrow to allow I − for further exchange. Interestingly, the fully substituted 3I-PAF-50 could be gained by exchange of I − ion with F-PAF-50. 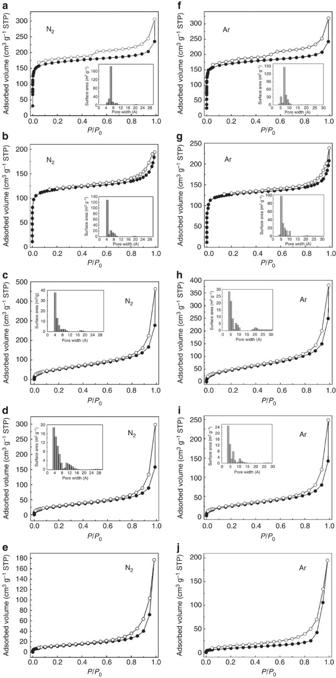Figure 2: Nitrogen adsorption isotherms. (a–j) Reversible nitrogen and argon gas adsorption isotherms for F-PAF-50 (a,f), Cl-PAF-50 (b,g), Br-PAF-50 (c,h), 2I-PAF-50 (d,i) and 3I-PAF-50 (e,j) measured at 77 K and 87 K, respectively. The inset is the profile of the pore size distribution calculated via NLDFT method. The binding energy of gas molecules on molecular segments was calculated by MS simulation environment employing grand canonical Monte Carlo simulation ( Supplementary Table 2 ). The values of binding energy follow an order of H 2 , O 2 , N 2 , CH 4 and CO 2 in small to large on each X-PAF-50. The high value of CO 2 would be due to a positive partial charge on the pyridinium groups promoted by the electron-withdrawing negative ion, leading to a polarizing binding environment, which could enhance the affinity for CO 2 owing to the dipole–quadrupole interactions [45] , [46] . N 2 sorption analysis The porous characteristics of PAFs were studied by N 2 sorption measured at 77 K and Ar sorption measured at 87 K, interpreted by the Brunauer-Emmet and Teller (BET) theory and non-localized density functional theory (NLDFT) method for consistency. As indicated in Fig. 2 , the typical type-I sorption isotherms of Cl-PAF-50 reveal its microporous properties. The surface area of Cl-PAF-50 was calculated to be 384 m 2 g −1 on the basis of the BET model; the pore size by NLDFT method is 5 Å with a narrow pore size distribution ( Fig. 2b ), which matches well with the simulated one. For other PAFs, N 2 sorption measurements showed similar type-I isotherms. However, the values of BET apparent surface areas of PAF-50 with different counter ions varied greatly ( Supplementary Table 1 ). F-PAF-50 possesses the highest BET surface area of 580 m 2 g −1 . In contrast, BET surface areas of Br-PAF-50 and 2I-PAF-50 are only 127 and 91 m 2 g −1 , respectively. Correspondingly, the major pore sizes and distributions for F-PAF-50 and Br-PAF-50 locate at around 7.0 and 4.4 Å, respectively. The pore sizes of 2I-PAF-50 are highly variable in distribution, except for the certain amount of pores centring at 3.9 Å, which is consistent with the theoretical diameter of existence of two I − ions and one Cl − ion per pore. For 3I-PAF-50, the pores are too narrow to be calculated by N 2 sorption ( Fig. 2e ). The hysteresis at the high relative pressures (0.6< P / P 0 <1.0) indicating the existence of mesoporosity and macroporosity, which can be attributed to the gaps between the particles. The adsorption behaviours and pore size distributions are further verified by the Ar sorption measured at 87 K. As observed in Fig. 2b , Ar sorption isotherms present similar behaviours with those of N 2 . BET surface areas of F-PAF-50, Cl-PAF-50, Br-PAF-50 and 2I-PAF-50 are 614, 337, 158 and 96 m 2 g −1 , respectively. Correspondingly, the major pore sizes and distributions for F-PAF-50, Cl-PAF-50, Br-PAF-50 and 2I-PAF-50 locate at around 6.7, 4.8, 4.5, and 3.8 Å, respectively. These results agree well with the ion content gained from ion-chromatography. Basically, the targeted adjustment of the pore size of PAFs can be realized through the exchange of the sterically hindered ions with different diameters. Figure 2: Nitrogen adsorption isotherms. ( a – j ) Reversible nitrogen and argon gas adsorption isotherms for F-PAF-50 ( a , f ), Cl-PAF-50 ( b , g ), Br-PAF-50 ( c , h ), 2I-PAF-50 ( d , i ) and 3I-PAF-50 ( e , j ) measured at 77 K and 87 K, respectively. The inset is the profile of the pore size distribution calculated via NLDFT method. Full size image Gases sorption analysis To distinguish the different pores in PAF-50 decorated with various counter ions, we obtained the adsorption isotherms of several light gases with different kinetic diameters, such as H 2 (2.89 Å), CO 2 (3.3 Å), O 2 (3.46 Å), N 2 (3.64 Å) and CH 4 (3.8 Å), by using a volumetric gas sorption apparatus. As shown in Fig. 3 , four PAFs demonstrated similar sorption isotherms towards same gases except O 2 . As to H 2 , a small rise at the low relative pressure ( P / P 0 <0.1) is observed and followed by a slow growth and eventual level off. The sorption volumes were 95.2, 67.5, 39.1 and 23.7 ml g −1 for F-PAF-50, Cl-PAF-50, Br-PAF-50 and 2I-PAF-50, respectively. With regard to other gases, these materials demonstrated a typical reversible sorption–desorption, and the uptakes for CO 2 are 74.6, 44.3, 25.2 and 6.8 ml g −1 , while about 35.1, 17.5, 5.2 and 2.3 ml g −1 of CH 4 are adsorbed on F-PAF-50, Cl-PAF-50, Br-PAF-50 and 2I-PAF-50 at 273 K and 1.0 atm, respectively. All the O 2 uptakes witness rapid rises at the initial stage, followed by the gradual rises as the pressure increases. The uptakes of PAFs were 265.7, 205.5, 91.8 and 69.1 ml g −1 for F-PAF-50, Cl-PAF-50, Br-PAF-50 and 2I-PAF-50, respectively. In the desorption stage, the hysteresis loops became broader obviously along with the decrease of pore sizes ( Fig. 3 ). 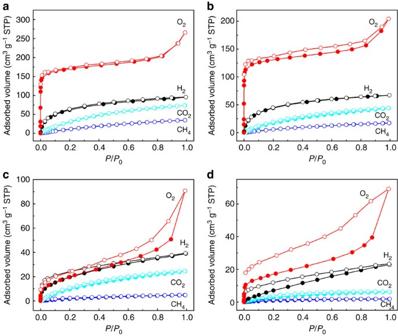Figure 3: Gas adsorption isotherms. (a–d) Gas adsorption isotherms of F-PAF-50 (a), Cl-PAF-50 (b), Br-PAF-50 (c) and 2I-PAF-50 (d) for H2and O2(P0=154 torr) at 77 K, CO2and CH4at 273 K. Figure 3: Gas adsorption isotherms. ( a – d ) Gas adsorption isotherms of F-PAF-50 ( a ), Cl-PAF-50 ( b ), Br-PAF-50 ( c ) and 2I-PAF-50 ( d ) for H 2 and O 2 ( P 0 =154 torr) at 77 K, CO 2 and CH 4 at 273 K. Full size image To better express the selectivity, the adsorption isotherms were calculated with Henry’s law ( Supplementary Note 1 ) that could reflect the affinity between the channel wall and the adsorbate [47] . As shown in Supplementary Table 3 , the selectivity becomes evidently higher as the pore size reduces. These results indicate that the PAF networks have strong affinity towards O 2 and N 2 molecules compared with H 2 , which are consistent with the previous theoretical calculation. As for O 2 , the large hysteresis implies the stronger interaction between the internal surface of 2I-PAF-50 and O 2 ( Supplementary Fig. 7 ). The most plausible explanation for this phenomenon lies in the probable confinement effect of oxygen in the pores, which is caused by the existence of bottlenecks along the galleries generated by reversible structure or by the introduction of anions at low temperature in narrow channels, thereby hindering the molecules motion [48] . This behaviour is analogous to the molecular sieving effect of zeolite 4A, which confirms the size-exclusive effect of PAF-50 in our study. The high levels of CO 2 uptake over CH 4 and their obvious hysteresis prove our hypothesis that the dipole–quadrupole interactions enhance the affinity for CO 2 with a high binding energy. Among the four samples, the sorption amount of the same gas declines sharply, which could be attributed to the fact that the saturation adsorption on the pore walls was easily reached along with the reduction of surface area. All these phenomena suggest that each PAF material may behave as a molecular sieve for the specific gas molecule according to their different interactions to the pore surfaces as well as their size-selective effect [49] . Gas-chromatographic separation To validate the sieving effect of the PAF-50 materials, the gas-chromatographic (GC) separation [6] , [50] at room temperature was employed, which could exhibit the differences in the diffusion rates of different components. The activated PAFs were packed into the columns (50 cm long × 2 mm internal diameter) as the stationary phase for GC separation and examined by several light gas mixtures in detail at room temperature using Ar as the mobile phase. In the GC separation experiments, F-PAF-50 exhibited a great ability in separating CO 2 , whose retention time is 6.44 min, from the mixture of other gases (H 2 , O 2 , N 2 and CH 4 ) with shorter retention time from 2 to 4 min ( Fig. 4a(i) ). As shown in Fig. 4a (ii–v) , these four gases could be separated from CO 2 during the binary mixture separation tests, including the mixture of CO 2 /H 2 , CO 2 /O 2 , CO 2 /N 2 and CO 2 /CH 4 . For Cl-PAF-50 and Br-PAF-50 column, the elution of both CO 2 and CH 4 are much slower than that of the H 2 , O 2 and N 2 mixture, thereby making CO 2 and CH 4 separable from the above mixture by turns. More importantly, according to Fig. 4b,c(ii–iv) , every single component can be separated adequately from the three-component gas mixture, such as CO 2 /CH 4 /H 2 , CO 2 /CH 4 /O 2 and CO 2 /CH 4 /N 2 . In the tests of 2I-PAF-50, in virtue of its 3.9 Å pores, the five-component gas mixture could be separated into three parts (H 2 , the mixture of N 2 /CH 4 and that of O 2 /CO 2 , as seen in Fig. 4d(i) ). As shown in Fig. 4d(ii–v) , 2I-PAF-50 can completely separate the three-component gas mixture such as H 2 /CH 4 /O 2 , H 2 /N 2 /CO 2 , H 2 /N 2 /O 2 and H 2 /CH 4 /CO 2 . In contrast, the commercial activated carbon whose pore size located at around 1 nm and the BET surface area is 840 m 2 g −1 ( Supplementary Fig. 8 ) is unable to separate the gas mixture ( Supplementary Fig. 9 ) with a broad retention time from 2 to 6 min. The pore size of F-PAF-50 is 7.0 Å, which is large enough for the five gases to pass through, but the unique selectivity might be dominated by the dipole–quadrupole interactions between CO 2 and the framework that enhance the affinity and prolong the retention time. 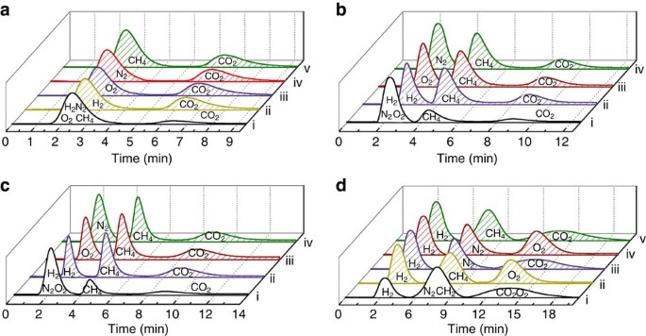Figure 4: GC chromatograms. (a–d) GC chromatograms on the F-PAF-50 (a), Cl-PAF-50 (b), Br-PAF-50 (c) and 2I-PAF-50 (d) packed open tubular column for separation of H2, N2, O2, CH4and CO2, respectively. (i) The separation behaviour of five-component mixture and (ii–v) the separation behaviours of representative mixture in detail. As for Cl-PAF-50 and Br-PAF-50, as seen in Supplementary Table 4 , the retention time of Br-PAF-50 for CH 4 is longer than that of Cl-PAF-50, which might demonstrate that the size-exclusive effect will become more evident as the pore size is close to the kinetic diameter of CH 4 . With regard to 2I-PAF-50, the nature of size exclusion is especially obvious. The selectivity is most likely caused by the size-exclusive effect between pores and gases. The kinetic diameter of H 2 is smaller than the pore diameter of 2I-PAF-50, whereas those of other four gases are close to its pore diameter. Thus, H 2 preferentially pass through the channels. Figure 4: GC chromatograms. ( a – d ) GC chromatograms on the F-PAF-50 ( a ), Cl-PAF-50 ( b ), Br-PAF-50 ( c ) and 2I-PAF-50 ( d ) packed open tubular column for separation of H 2 , N 2 , O 2 , CH 4 and CO 2 , respectively. (i) The separation behaviour of five-component mixture and (ii–v) the separation behaviours of representative mixture in detail. Full size image To better understand the interaction, H 2 , O 2 , N 2 and Ar sorption isotherms were measured at 273 K and 1 atm ( Supplementary Fig. 10 ). As observed, each X-PAF-50 exhibited the similar gas sorption amount and sorption behaviour to H 2 , N 2 and Ar. As to O 2 , there is still a large hysteresis implying the stronger interaction between the internal surface of 2I-PAF-50 and O 2 at 273 K. These results also verify that the gas separation is due to the effect of pore sizes irrespective of the surface area. Total separation Encouraged by the polymeric sieves effect of the above PAFs to specific multi-component gas mixture, experiment was carried out to separate the total five-component gas mixture. Combining the capability of Cl-PAF-50 to separate CH 4 and CO 2 from gases of H 2 /O 2 /N 2 and that of 2I-PAF-50 to isolate H 2 , N 2 and O 2 , the columns of Cl-PAF-50 with 120 cm × 2 mm and 2I-PAF-50 with 50 cm × 2 mm were connected for the total separation. As shown in Fig. 5 , the connective column could separate the mixtures of the five-component gas mixture efficiently with retention times at 6.05, 10.37, 19.24, 28.26 and 37.54 min for H 2 , N 2 , O 2 , CH 4 and CO 2 , respectively. The demonstrated PAF materials promise a potential application in gas separations with high efficiency. 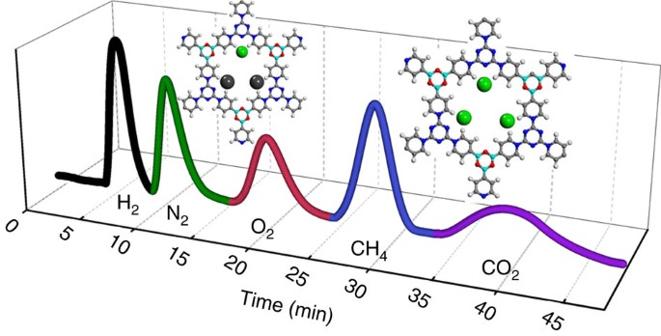Figure 5: Total separation. GC chromatograms on the Cl-PAF-50 and 2I-PAF-50 connective column for separation of H2, N2, O2, CH4and CO2mixture. Figure 5: Total separation. GC chromatograms on the Cl-PAF-50 and 2I-PAF-50 connective column for separation of H 2 , N 2 , O 2 , CH 4 and CO 2 mixture. Full size image In summary, through a feasible ion exchange method, a family of positively charged quaternary pyridinium-type PAFs (X-PAF-50, X=F, Cl, Br, I) have been prepared and their pores can be tuned systematically at the angstrom scale from 3.4 to 7 Å. These PAFs exhibit distinctive molecular sieving effect to separate multi-component gas mixtures. The results of this research have important significance on the practical design and preparation of porous materials for gas separations. Besides, by combining their specific separation merits, the total five-component gas mixture can be separated completely by turns. The great operation ease and technical flexibility of PAFs hold immense promise in practical and commercial applications as polymeric sieves. Materials All starting materials, organic solvents and polymers were purchased from commercial suppliers and used without further purification unless otherwise noted. All reactions were performed under a purified nitrogen atmosphere. Synthesis of Cl-PAF-50 Cyanuric chloride (11.8 g, 60 mmol) and 4-pyridinylboronic acid (22.13 g, 180 mmol) were added into 800 ml toluene and degassed by three repetitions of freezing, pump and thawing procedure. The mixture was heated at 120 °C for 36 h. After cooling to room temperature, the resulting precipitates were filtered and washed with CHCl 3 (90 ml), THF (90 ml) and toluene (90 ml) for five times each, followed by drying in vacuo at room temperature. The Cl-PAF-50 was obtained in the form of grey-purple powder (20.7 g, 70% yield). Preparation of the substituted PAFs Activated Cl-PAF-50 (1.665 g, containing 10 mmol Cl − ) was washed with ethanol three times until no free Cl − was released, and then dispersed the powder in anhydrous ethanol (50 ml). The solution of corresponding tetrabutylammonium salts (tetrabutylammonium fluoride, tetrabutylammonium bromide or tetrabutylammonium iodide) in anhydrous ethanol (1 mol l −1 , 15 ml) was then added to the above mixture. After the mixture was stirred for 24 h, the residue was filtered. Repeated the above step six times, the precipitate was washed with anhydrous ethanol (50 ml) five times and then afforded the goal product. Preparation of 3I-PAF-50 Activated F-PAF-50 (1.50 g) was dispersed in anhydrous ethanol (50 ml). The solution of tetrabutylammonium iodide in anhydrous ethanol (1 mol l −1 , 15 ml) was then added to the above mixture. After the mixture was stirred for 24 h, the residue was filtered. Repeated the above step eight times, the precipitate was washed with anhydrous ethanol (50 ml) five times and then afforded the goal product. It is noteworthy that the whole process must be operated in completely anhydrous environments. Measurements TGA was performed using a Netzch Sta 449c thermal analyzer system at the heating rate of 10 °C min −1 in air atmosphere. FT-IR spectra were measured using a Nicolet Impact 410 Fourier transform infrared spectrometer. Elemental analysis was carried out on a Perkin-Elmer 240C elemental analyzer. N 2 adsorption isotherms were measured on a Micromeritics ASAP 2010M analyzer. X-ray diffraction patterns were obtained on a Riguku D/MAX2550 diffractometer using CuKα radiation, 40 kV, 200 mA with scanning rate of 0.3° /min (2θ). TEM was implemented on a JEOL JEM 3010 with an acceleration voltage of 300 kV. SEM was performed on a JEOS JSM 6700. The content of the halide ions were performed by ion-chromatographic analyzer ICS-900. The models of PAFs are constructed by the use of the MS simulation environment employing MS Visualizer. GC separation was performed with a SP-2100A GC system equipped with a thermal conductivity detector. GC separation measurements The stainless steel tube (50 cm long × 2 mm internal diameter) was positioned vertically against the floor. The lower end of the tube was blocked by glass wool and wrapped with a rubber plug. About 1.0 g of PAF powders were poured into the column; then the column was stirred every once in a while to ensure no void left. Argon (99.999%) was used as the carrier gas and was driven at the inlet pressure of 40 kPa. Before GC experiments, the column was activated at 120 °C with Ar flow for 24 h. Then, 1.0 ml of equimolar mixtures was injected through an automatic gas-sampling valve. How to cite this article: Yuan, Y. et al . Porous aromatic frameworks with anion-templated pore apertures serving as polymeric sieves. Nat. Commun. 5:4260 doi: 10.1038/ncomms5260 (2014).